Single-mode tunable laser emission in the single-exciton regime from colloidal nanocrystals Whispering-gallery-mode resonators have been extensively used in conjunction with different materials for the development of a variety of photonic devices. Among the latter, hybrid structures, consisting of dielectric microspheres and colloidal core/shell semiconductor nanocrystals as gain media, have attracted interest for the development of microlasers and studies of cavity quantum electrodynamic effects. Here we demonstrate single-exciton, single-mode, spectrally tuned lasing from ensembles of optical antenna-designed, colloidal core/shell CdSe/CdS quantum rods deposited on silica microspheres. We obtain single-exciton emission by capitalizing on the band structure of the specific core/shell architecture that strongly localizes holes in the core, and the two-dimensional quantum confinement of electrons across the elongated shell. This creates a type-II conduction band alignment driven by coulombic repulsion that eliminates non-radiative multi-exciton Auger recombination processes, thereby inducing a large exciton–bi-exciton energy shift. Their ultra-low thresholds and single-mode, single-exciton emission make these hybrid lasers appealing for various applications, including quantum information processing. Research in developing lasers based on semiconductor nanocrystals for applications, such as telecommunications, optical interconnects and quantum information processing, has experienced significant growth over the past decade. This activity has resulted in the demonstration of a whole range of sources, including ultra-short (~100 fs) pulse lasers with a few kHz narrow linewidths [1] , operating with GHz-repetition rates [2] , and ultra-low timing jitter as well as single-photon sources based on photonic crystals [3] , micropillars [4] and nanowires [5] . Although epitaxial growth techniques that are compatible with complementary metal-oxide-semiconductor technology represent an established approach to produce self-assembled nanocrystals for photonic devices, the use of wet-chemistry methods has emerged in recent years as a simpler and cost-effective fabrication alternative. Attractive features of chemically synthesized nanocrystals include the ease of control over their size, shape, compositional and surface chemical properties, and the wealth of possibilities for their incorporation into micro- and nanocavities, photonic crystals, feedback schemes and material matrices. Among the different types of colloidal nanocrystals, core/shell heterostructures, consisting of a quantum dot (core) embedded in a nanoshell, predominantly with spherical and, more recently, with linear [6] branched [7] and platelet [8] , [9] geometries, have been under vigorous research investigation for the development of microlasers [10] , [11] , [12] , [13] , [14] , [15] , [16] , [17] , [18] , [19] , fundamental studies of light–matter interactions and solid-state cavity quantum electrodynamic effects [20] , [21] , where the end goal is to realize functions, such as entanglement of distinguishable quantum systems and controlled coherent coupling. The potential of these nanostructures in lasing applications with respect to bare quantum dots relies on their ability to reduce surface/interface defects and suppress non-radiative Auger recombination effects, as it has been demonstrated using different approaches, involving the use of shells with large thickness or gradual composition, or engineering of the carrier wavefunctions in the volume of the nanostructure [22] , [23] , [24] , [25] . This provides prospects for realization of lasing in the single-exciton regime, involving the recombination of a single electron–hole pair (exciton). Optical gain in bare quantum dots instead relies on multi-exciton states and experiences a fast decay resulting from non-radiative Auger recombination triggered by quantum-confinement-enhanced Coulombic carrier–carrier interactions [26] , [27] . Furthermore, in core/shell nanocrystals the encapsulating shell protects the core from photodegradation, thereby ensuring significantly higher photoluminescence (PL) quantum yields [28] , [29] . An effective approach to circumvent the detrimental Auger recombination effect and obtain single-exciton emission has been recently demonstrated in a vertical cavity surface emitting lasing configuration using core/shell, dot/dot CdSe/Zn 0.5 Cd 0.5 S nanocrystals with type-I conduction band (CB) alignment [18] as a gain medium. The alloyed shell in these structures ensured a smooth profile for the confinement (interfacial core/shell) potential, which has been associated with lower Auger recombination rates, resulting from the attenuation of high-frequency components in the ground-state hole wavefunction [30] , [31] . The supressed Auger rates allowed for low lasing thresholds for an ensemble averaged number of excitons of ›N‹ <1 (ref. 18 ). Here we demonstrate for the first time single-mode, single-exciton, tunable laser emission from an ensemble of colloidal type-II CdSe/CdS core/shell nanorods on a silica microsphere. Core/shell nanocrystals with type-II bandgap alignment at the core/shell interface have been extensively studied over recent years, as they represent another promising route for realizing single-exciton lasers [32] , [33] , [34] . The CBs of the CdSe core and the CdS shell in our nanorods are engineered such that the lowest energy states for holes and electrons reside in the core and shell, respectively. The Coulombic repulsive forces that developed along the length of the shell upon optical excitation result in the development of electric field within their volume, which induces a Stark shift of the absorption wavelength with respect to the emission one and allows for single-exciton lasing. One advantage of the dot (core)/rod (shell) architecture adopted here, which represents the simplest extension to the basic spherical core/shell geometry [6] , is that it provides additional options for shape engineering and, in turn, for manipulation of the carriers’ wavefunction distributions, and the optical and electronic properties of the nanocrystals [35] , [36] , [37] , [38] . Furthermore, nanocrystals with elongated geometries exhibit higher absorption coefficients compared with their spherical counterparts, which allows them to act in a way as antennas for optical excitation [7] . Hybrid lasers with whispering-gallery-mode microresonators The colloidal CdSe/CdS nanorods were synthesized by the seeded-growth approach [29] . They could produce PL quantum yields as high as 65% [29] , and had an effective refractive index of n nc =2.5 at λ =610 nm, a wavelength that corresponds to their ensemble PL peak. Their structure was asymmetric, consisting of a spherical, optically active CdSe core with a diameter of 4.0±0.7 nm embedded in one end of the elongated (28±2 nm) CdS shell. Because of its large absorption cross-section, the latter acts as a sensitizer by efficiently absorbing pump light and conferring the photoexcitation to the CdSe core. As the valence band (VB) offset between the two materials is 0.78 eV [39] , holes experience a three-dimensional confinement within the core. On the other hand, the offset of their CBs depends on the aspect ratio of the nanorods and their growth conditions, ranging from −0.3 to 0.3 eV (refs 39 , 40 , 41 ). The microspheres were produced by CO 2 laser thermal processing of fibre tapers (see Methods) to which they remained attached after the completion of the fabrication process. They had diameters from 8 to 40 μm, measured Q -factors in excess of 10 8 and were coated with a thin layer of nanorods by immersion in a toluene solution of the latter. The density of the nanorods attached on the microsphere surface was controlled by varying their concentration in the solution, the immersion time and the withdrawal speed of the microspheres from the solution. A schematic of the experimental setup and an image of a typical microsphere used in our work are shown in Figs 1 and 2a , respectively. The spheres were pumped at wavelengths ~400 nm with a tuneable frequency-doubled Ti:sapphire amplifier, operating at 250 KHz and emitting 180-fs-short pulses with a linewidth of 5 nm. The pump light was evanescently coupled to the microsphere resonators using tapered optical fibres with adiabatic transitions, drawn from single-mode fibres at 405 nm (see Methods). This method ensures efficient incoupling and outcoupling of the pump and laser beam, respectively, as well as selectivity in the excitation of the modes [42] , [43] . 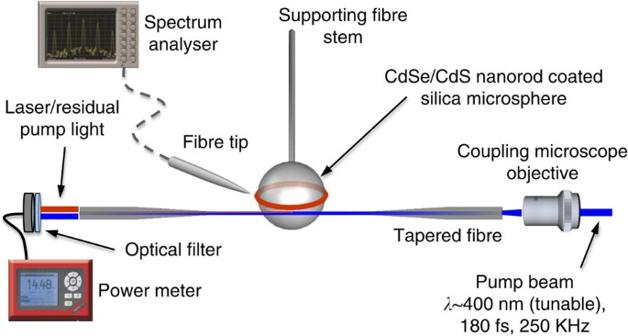Figure 1: Experimental setup for demonstration of lasing in CdSe/CdS colloidal nanorods. Self-assembled nanorods on silica microspheres were excited by bringing the evanescent field of the fibre taper in the proximity of the microsphere, thereby establishing an overlap of the fundamental optical mode of the taper with the WGMs. The position of the taper relative to the microsphere was controlled by high-resolution, three-axis nano-positioning stages, allowing for tuning of the phase-matching conditions and optimization of coupling. The tip could be brought into contact with the sphere and then moved on the surface along a meridian to the desired plane. Emission spectra were recorded with an optical spectrum analyser. The absorbed pump power was measured as the difference of the power launched into the taper and that transmitted after the taper. To obtain the power of the laser signal that was evanescently coupled from the microsphere into taper, unabsorbed pump light transmitted through the latter was removed from the laser emission light with a suitable filter. Figure 1: Experimental setup for demonstration of lasing in CdSe/CdS colloidal nanorods. Self-assembled nanorods on silica microspheres were excited by bringing the evanescent field of the fibre taper in the proximity of the microsphere, thereby establishing an overlap of the fundamental optical mode of the taper with the WGMs. The position of the taper relative to the microsphere was controlled by high-resolution, three-axis nano-positioning stages, allowing for tuning of the phase-matching conditions and optimization of coupling. The tip could be brought into contact with the sphere and then moved on the surface along a meridian to the desired plane. Emission spectra were recorded with an optical spectrum analyser. The absorbed pump power was measured as the difference of the power launched into the taper and that transmitted after the taper. To obtain the power of the laser signal that was evanescently coupled from the microsphere into taper, unabsorbed pump light transmitted through the latter was removed from the laser emission light with a suitable filter. 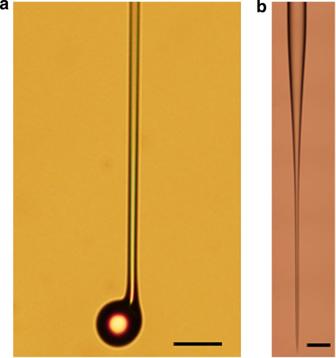Figure 2: Microsphere template and optical fibre tip images. Optical microscope images of (a) a silica microsphere with a diameter of ~30 μm, used as a template for the CdSe/CdS quantum rods and (b) an optical fibre tip with a diameter of 50 nm and a 2-mm-long taper transition used to collect signals from the CdSe/CdS nanocrystal/silica microsphere hybrid resonators. Scale bars, (a) 30 μm; (b) 125 μm. Full size image Figure 2: Microsphere template and optical fibre tip images. Optical microscope images of ( a ) a silica microsphere with a diameter of ~30 μm, used as a template for the CdSe/CdS quantum rods and ( b ) an optical fibre tip with a diameter of 50 nm and a 2-mm-long taper transition used to collect signals from the CdSe/CdS nanocrystal/silica microsphere hybrid resonators. Scale bars, ( a ) 30 μm; ( b ) 125 μm. Full size image To measure their optical power and record their spectra, the laser signals were collected by the same taper used for pumping. In cases when the laser output characteristics of the hybrid source were studied, a probe fibre tip [44] ( Fig. 2b ) with a diameter of ~50 nm, a size that ensured sufficient resolution was employed for in-situ monitoring of the laser spectra (see Methods for fabrication details). To enhance pump efficiency and prevent excitation of whispering-gallery modes (WGMs) with high radial index, n , phase-matching of the propagation coefficients between the propagating fundamental mode in the taper and a fundamental WGM in the microsphere (that is, matching of the spatial period of the optical waves in both the taper and microsphere resonator, and hence constructive interference) was established by suitably choosing the size of taper diameter (typically from 1 to 2 μm) with respect to that of the sphere [42] . Establishing phase matching of the fundamental taper mode to a given WGM also improved the coupling ‘ideality’ defined as the ratio of power coupled to a desired mode divided by the power coupled or lost to all modes [43] . Because of the large absorption by the nanorods at the pump wavelength and, hence, the large round-trip loss in the microsphere resonator, any mode other than the fundamental that may have been excited by the fraction the pump power that was not transferred to fundamental WGMs would be eliminated. 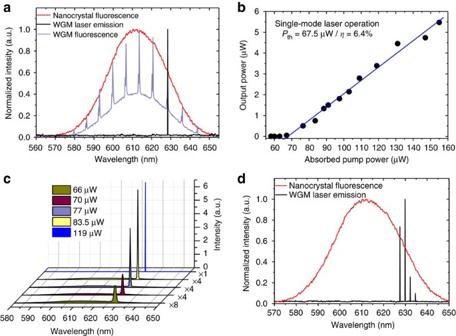Figure 3: Fluorescence and laser emission characteristics. (a) Single-mode, single-exciton laser (black line) and WGM fluorescence (blue line) emission spectra obtained from a 9.2-μm-diameter hybrid sphere by pumping an equatorial ring region. In the background, the fluorescence produced by the ensemble of CdSe/CdS nanorods attached to the sphere is also presented (red line). (b) Output power as a function of absorbed pump power for the single-mode, single-exciton laser operation of a 9.2-μm-large hybrid microsphere. (c) Evolution of the laser-emission spectral line for different absorbed pump powers near the lasing threshold. (d) Laser emission spectrum obtained from a microsphere with a diameter of 29.4 μm by pumping at its equatorial zone. The distance between the modes (~2.4 nm) corresponds to the FSR of the sphere. Figure 3a shows the laser spectrum for the single WGM operation at 628.32 nm of a microsphere with a diameter of 9.2 μm, along with the inhomogeneously broadened fluorescence spectrum from an ensemble of nanocrystals and the PL emission spectrum from the hybrid microsphere. The latter exhibits a modulation by a number of peaks with the characteristic WGM distribution. The laser spectrum was obtained by resonantly pumping a fundamental WG pump mode with , with m and l being the azimuthal and polar numbers, respectively, above an absorbed pump power of 100 μW. Such modes, with low n numbers, have very small volumes and are confined to the equatorial ring of the sphere (defined as the area parallel to the taper fibre axis perpendicular to the stem) close to its surface [45] . They were identified by a dip observed in the transmission through the taper when the pumping wavelength was tuned. The laser line corresponds to the single-exciton transition and its full-width at half-maximum (FWHM) value of Δλ =0.06 nm suggests a Q -factor value of λ / Δλ ~10 4 for the hybrid cavity. This lower value, with respect to the uncoated sphere, is attributed to the surface roughness introduced by the gain medium and the associated scattering loss at the boundaries with the silica microsphere and the surrounding air. Losses from the presence of the fibre may also have contributed to the deterioration of the Q -factor, as experiments were conducted near the overcoupled regime. Parameters that are crucial for achieving single-mode laser emission from the hybrid microsphere are the bandwidth of the pump pulse at ~400 nm, the microsphere size, and the establishment of phase-matching pumping conditions. Microspheres with sufficiently small size have a free-spectral range (FSR) that is comparable to or larger than the bandwidth of the pulse, which allows for spatially selective excitation of a single mode. Phase matching of this mode with the pump taper mode ensures maximum optical pump power transfer. In this case, the optical power transferred to other non-phase-matched modes is significantly smaller and insufficient to produce lasing because of large absorption of the pump wavelength by the microsphere and the associated high losses in the resonator. Figure 3: Fluorescence and laser emission characteristics. ( a ) Single-mode, single-exciton laser (black line) and WGM fluorescence (blue line) emission spectra obtained from a 9.2-μm-diameter hybrid sphere by pumping an equatorial ring region. In the background, the fluorescence produced by the ensemble of CdSe/CdS nanorods attached to the sphere is also presented (red line). ( b ) Output power as a function of absorbed pump power for the single-mode, single-exciton laser operation of a 9.2-μm-large hybrid microsphere. ( c ) Evolution of the laser-emission spectral line for different absorbed pump powers near the lasing threshold. ( d ) Laser emission spectrum obtained from a microsphere with a diameter of 29.4 μm by pumping at its equatorial zone. The distance between the modes (~2.4 nm) corresponds to the FSR of the sphere. Full size image Figure 3b shows the laser output characteristics as a function of absorbed pump power for the single WGM operation of the microsphere, indicating a lasing threshold of 67.5 μW and a maximum output power of 5.5 μW for 155 μW of absorbed power, which corresponds to a slope efficiency of η =6.4%. The evolution of the emission line for different absorbed pump powers around the lasing threshold of the hybrid source is displayed in Fig. 3c , exhibiting a progressive spectral narrowing of the linewidth with increasing pump power from ~1.3 nm (FWHM) just below threshold at 66 μW, to 0.06 nm at absorbed pump powers near and in excess of 119 μW. Furthermore, a significant increase in the emission peak intensity above threshold can be observed, which follows a linear behaviour as shown in Fig. 3b . Microspheres with larger diameters produced a multi-mode laser emission due to the smaller FSR, Δ λ FSR , in between the modes with adjacent l indices. Figure 3d shows a laser-emission spectrum obtained from a microsphere with a diameter of 29.4 μm by pumping at the equatorial zone. The lasing modes in the spectrum appear at wavelengths separated by a distance of 2.4 nm, which is very close to the value of Δ λ FSR =2.375 of the hybrid microsphere derived from the equation [46] where λ L =628.32 nm is the emission wavelength of the first mode, n s =1.47 is the refractive index of the silica microsphere, whereas R H =14.7 μm is the radius of the hybrid sphere, which was assumed to be equal to that of the silica template. Laser emission by single-exciton and bi-exciton transitions The modality of the laser emission can also be tuned by varying the coupling conditions and the optical pump power. Hence, evanescent coupling of the pump beam into the resonator away from its equatorial zone results in a multi-mode laser emission as shown in Fig. 4a , where, apart from the laser line at 628.32 nm, a second laser line emerges at lower wavelengths near 592.6 nm. Non-equatorial pumping effectively invalidates the aforementioned conditions for single modality, as it leads to the excitation of a number of modes with different radial and azimuthal numbers, thereby inducing multi-mode lasing. This multi-mode behaviour becomes evident by moving the tapered fibre by a distance of approximately half the width of the tapered fibre (that is of the order of 0.5 μm) away from the equator. 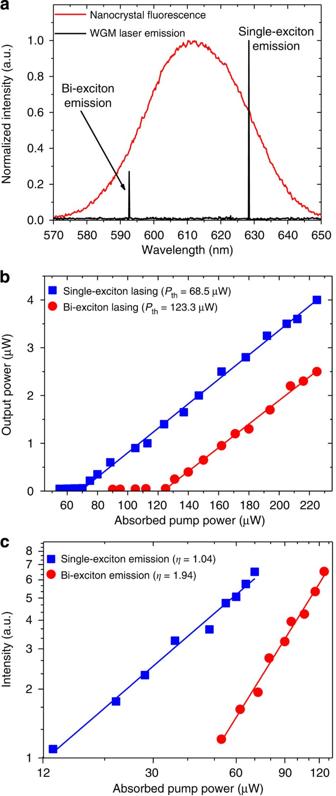Figure 4: Laser operation in the single-exciton and bi-exciton regimes. (a) Laser spectrum obtained for 130 μW of absorbed power by non-equatorial pumping, showing emission on the single- and bi-exciton transitions; (b) Output characteristics of the single-exciton and bi-exciton laser emission; (c) input–output characteristics of the single-exciton and bi-exciton emission in the preleasing regime, exhibiting slopes of ~1 and ~2, respectively. Figure 4b shows the output characteristics of the two laser lines, revealing pump power thresholds of 68.5 and 123.3 μW for the low-energy and high-energy transitions, respectively. The data points were obtained by using suitable wavelength cut-off filters to isolate the laser emission of each transition. The dependency of the optical power of the two lines on absorbed pump power in the pre-lasing (linear) regime is displayed in a log–log plot in Fig. 4c . The slope efficiencies of η ≈1 and 2 derived suggest a linear and a quadratic dependence for the transitions in the low- and high- energy spectral area, which are typical of single- and bi-excitonic gain mechanisms, respectively. Furthermore, the threshold of the laser emission at 592.6 nm is approximately twice as high as that at 628.32 nm, thereby providing an additional proof of their bi-excitonic and single-excitonic nature of the corresponding transition, respectively. Figure 4: Laser operation in the single-exciton and bi-exciton regimes. ( a ) Laser spectrum obtained for 130 μW of absorbed power by non-equatorial pumping, showing emission on the single- and bi-exciton transitions; ( b ) Output characteristics of the single-exciton and bi-exciton laser emission; ( c ) input–output characteristics of the single-exciton and bi-exciton emission in the preleasing regime, exhibiting slopes of ~1 and ~2, respectively. Full size image As an additional verification of the assignment of the laser lines in Fig. 4a to the single-exciton and bi-exciton CdSe transitions, we calculated their energies. To this end, we derived the wavefunctions ψ e (electron) and ψ h (hole) from the Schrödinger equations by using an iterative process involving the effective mass approximation method, and taking into account the Coulomb interaction (see Methods). Effective mass approximation has emerged over the years as a reliable approach for reproducing the energy spectra of confined excitons in semiconducting nanocrystals, by successfully addressing the problem of choosing the actual electrical potential felt by each carrier in the corresponding Schrödinger equations [47] , [48] . In this process, we first sequentially varied the CB offset and the nanorod diameter following the Hartree self-consistent potential approach [49] so as to match the single-exciton emission wavelength with that of the experimental line at 628.32 nm. In this process, the nanorod length was maintained fixed at a value of 28 nm, as this parameter has insignificant impact on the confinement effect within the limits of the deviation (±2 nm) from this value associated with the nanocrystal synthesis process. As a result, we obtained very good agreement by assuming an offset value of −0.09 eV and a diameter of 4.34 nm; the energy eigenvalues derived for the electron and the hole with respect to the bottom of the conduction and VBs of CdSe were 0.14876, eV and 0.14349, eV, respectively, thereby suggesting single-exciton lasing at 628.6 nm. 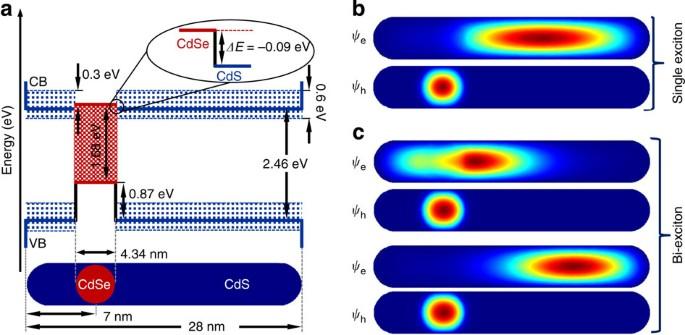Figure 5: Electronic structure and calculated wavefunctions in CdSe/CdS core/shell nanorods. (a) Schematics of a CdSe/CdS dot/rod nanocrystal along with the interfacial band alignment of the CdSe and CdS constituent materials. The core diameter (4.34 nm) and the CB offset (−0.09 eV, inset) correspond to the values adopted for the calculation of the electronic wavefunctions and lasing wavelengths. The values of the VB offset (0.87 eV) along with those of the bandgaps for CdSe (1.68 eV) and CdS (2.46 eV) are also shown. The blue shadowed area indicates the range of potential values for the CB offset. (b,c) Calculated wavefunctions for the electrons (ψe) and holes (ψh) for the laser emission in (b) the single-exciton regime at 628.6 nm, exhibiting mixed carrier dimentionality and small overlap, and (c) the bi-exciton regime at 593.3 nm, indicating that for the first exciton the hole/electron wavefunctions are localized in/near the core, and for the second exciton they are separated and are located in the core and the shell, respectively. Figure 5a displays a schematic of the nanorod along with a band alignment diagram at the heterointerface between its core and shell, indicating the values adopted for the core diameter and the CB offset in our calculations. The calculated wavefunctions are displayed in Fig. 5b , showing spatial separation between the hole and the electron charge densities with the holes remaining confined to the CdSe core and the electrons being delocalized in one dimension over the entire nanostructure. Such carrier distributions are typical of type-II core/shell nanocrystals, and result in very small overlaps [2] of their wavefunctions. Next, we calculated the wavefunction distributions and emission wavelength for the bi-exciton, by adopting the same values for the offset and the nanorod size used for our calculations in the single-exciton regime. Figure 5c shows the calculated wavefunctions, wherein one exciton there is a zero charge density, whereas in the other same-sign charges are spatially well separated. The calculated energy eigenvalues for the pairs of electrons and holes are (0.15162 and 0.15363, eV) and (0.19835 and 0.19835, eV), respectively. These values, which are unique within the size limits of the nanocrystals used in our experiment yield bi-exciton laser emission at 593.3 nm, which is very close to the spectral line observed at 592.6 nm. Figure 5: Electronic structure and calculated wavefunctions in CdSe/CdS core/shell nanorods. ( a ) Schematics of a CdSe/CdS dot/rod nanocrystal along with the interfacial band alignment of the CdSe and CdS constituent materials. The core diameter (4.34 nm) and the CB offset (−0.09 eV, inset) correspond to the values adopted for the calculation of the electronic wavefunctions and lasing wavelengths. The values of the VB offset (0.87 eV) along with those of the bandgaps for CdSe (1.68 eV) and CdS (2.46 eV) are also shown. The blue shadowed area indicates the range of potential values for the CB offset. ( b , c ) Calculated wavefunctions for the electrons ( ψ e ) and holes ( ψ h ) for the laser emission in ( b ) the single-exciton regime at 628.6 nm, exhibiting mixed carrier dimentionality and small overlap, and ( c ) the bi-exciton regime at 593.3 nm, indicating that for the first exciton the hole/electron wavefunctions are localized in/near the core, and for the second exciton they are separated and are located in the core and the shell, respectively. Full size image To evaluate the potential of the gain medium to produce optical gain by single-exciton states without any involvement of multi-excitons, we have derived the gain threshold › N th ‹ expressed in terms of the average number of excitons per nanocrystal [33] : where Δ xx =119 meV represents the spacing between the single- and bi-exciton line at 626.32 nm and at 592.6 nm, respectively, and Γ is the emission linewidth of a single nanocrystal at room temperature. For the latter, we have adopted an upper value of Γ =65 meV, which was recorded for the emission of a single CdSe/CdS core/shell tetrapod-shaped nanocrystal with an arm-length of 30 nm [50] at room temperature. From equation (2), we obtain a value of › N th ‹=0.675, which is well below the theoretical value of › N th ‹=1 for bi-exciton gain in homogeneously broadened type-I nanocrystals and very near to that of ideal type-II nanocrystals (› N ‹=2/3) [33] . The latter are associated with considerably larger Δ xx values with respect to the transition linewidth, thereby allowing for the elimination of absorption losses and, hence, for optical gain from single-exciton states. Wavelength-tuneable laser emission Tuning the emission from spherical microcavities has been realized either by modulating the pump power, thereby exploiting the thermo-optical effect of the active material [51] , or by using external heating sources [52] , or with the application of pressure or strain [53] . Although the tuning ranges achieved with the strain method can even approach the frequency separation between adjacent resonance peaks of the WGMs [53] , thereby exceeding those obtained by temperature variation, the latter has the attraction of enhanced accuracy of control over the emission wavelength. In this work, the lasing wavelength, λ L , was tuned by heating the 9.2-μm large hybrid microsphere with 3.5-μm pulses of 200 fs duration and 80 MHz repetition rate from a tunable femtosecond laser, which were directed onto the microsphere by a microscope objective. The optical power of the infrared laser beam was raised in successive steps, and for each step the wavelength of the pump laser was modulated so as to excite resonant WGMs that were gradually shifted in wavelength due to the temperature elevation. Throughout these experiments, the evanescently coupled power was maintained constant at 100 μW. The laser spectrum was recorded for each pump power setting, indicating a maximum wavelength red shift of 2.1 nm within the available power range of 60 mW ( Fig. 6a ), which corresponds to ~30% of the FSR at λ L . 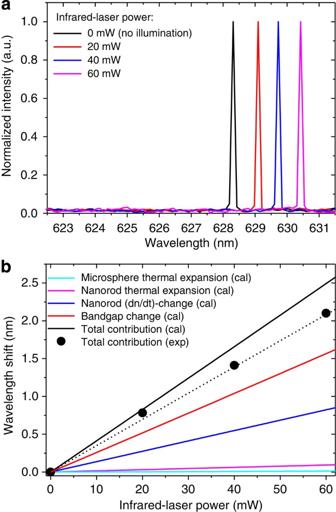Figure 6: Tunable laser emission from CdSe/CdS nanorods. (a) Laser emission obtained from a 9.2-μm large hybrid microsphere for different output powers of the infrared laser that served as a heating source. (b) Calculated (black line) and measured (symbols) red shift of the lasing wavelength as a function of output power of the infrared laser. The dotted line is a guide for the eye for the experimental results. The coloured lines represent the calculated contributions of the thermal expansion of the silica microsphere (cyan) and the CdSe/CdS nanorods (purple), as well as of the nanorods’ thermo-optic coefficient (blue) and the change of their bandgap size (red). Figure 6: Tunable laser emission from CdSe/CdS nanorods. ( a ) Laser emission obtained from a 9.2-μm large hybrid microsphere for different output powers of the infrared laser that served as a heating source. ( b ) Calculated (black line) and measured (symbols) red shift of the lasing wavelength as a function of output power of the infrared laser. The dotted line is a guide for the eye for the experimental results. The coloured lines represent the calculated contributions of the thermal expansion of the silica microsphere (cyan) and the CdSe/CdS nanorods (purple), as well as of the nanorods’ thermo-optic coefficient (blue) and the change of their bandgap size (red). Full size image As at λ =3.5 μm the nanorods are transparent, the observed shift is expected to result from a temperature-induced increase in the size of the absorbing silica microsphere; other contributions originate from changes of the thermo-optic coefficient ( dn nc / dT =1 × 10 −4 K −1 ), bandgap energy (Δ E g ) and the nanorods size due to a temperature rise induced by heat conduction from the microsphere. The effect of these factors on the tuning range of the lasing wavelength Δλ L can be described by: where Δ T is the temperature rise in the hybrid microsphere, α s =5.5 × 10 −7 K −1 and α nc =4.5 × 10 −6 K −1 are the thermal expansion coefficients of silica and the nanorods, respectively, and Δ λ bg represents the wavelength shift resulting from Δ E g . For α nc and dn nc / dT , we adopted the values of the bulk CdS crystal. To investigate the consistency of the experimentally obtained tuning range, we estimated Δ T and Δ λ bg , and subsequently calculated Δ λ L from equation (3). To derive an analytical expression for Δ T , we assumed that the impact of the thin nanorod layer on the temperature of the laser-heated silica sphere is negligible, meaning that they both have effectively the same temperature (see Methods). The microcavity can be therefore considered as a solid consisting of a single material (silica), which is heated by a focused laser beam in the surrounding air. As the latter is transparent at the illumination wavelength, it is expected to reduce the temperature of the hybrid microsphere. Following an approach used to address a similar problem [54] based on solving the heat equation, we derived by adopting appropriate boundary conditions (see Methods) for Δ T the expression: where κ α =2.6 × 10 −2 mW m −1 K −1 and κ s =1.38 × 10 −3 mW m −1 K −1 are the thermal conductivities of the air and silica, respectively, P o is the illumination laser power and is the heat transferred from the sphere to the air. The term P abs =0.65 represents the optical power fraction absorbed by the silica, with R fr being the Fresnel reflection at the air/nanorods and nanorods/silica interfaces given by: with n α =1 being the refractive index of the air. In calculating Δ T in equation (4), one has to consider that due to the Gaussian beam profile and the spherical shape of the microcavity, parts of the beam impinging on the sphere at angles that deviate considerably from the normal experience high reflections and, therefore, have a negligible contribution to Δ T . As a satisfactory approximation, we assumed that only the optical power included within the FWHM of the beam, that is 50% of the total power, contributes effectively to the temperature elevation. To account for this effect, we introduced the term P g =0.5 in equation (4), which then yields for the maximum available infrared-laser power of 60 mW a value of Δ T =32.7 K. Returning to equation (3), we calculated Δ λ bg from the expression where the wavelength that corresponds to the bandgap energy λ bg is set equal to λ L . For the calculated temperature increase of Δ T =32.7 K, Δ E g can be derived from with β =216 K, α =1.8 × 10 −4 eV/K and E g (0)= 2.13 eV being correspondingly the Debye temperature, a temperature constant and the bandgap at 0 K. Figure 6b shows the calculated effect of each of the four individual parameters and their combined impact on Δ λ together with the experimentally obtained wavelength shifts. The latter are smaller than the calculated ones, arguably because of a weaker absorption of the heating beam from the microsphere than that assumed and/or an imperfect alignment of the infrared-laser beam with respect to the microsphere, meaning that in reality the Δ T induced was about 28 K, as it can be derived from equation (4). It is worth noting that for Δ T =32.7 K, the increase in the nanorod size would not exceed 0.01 nm, which precludes any contribution to the laser wavelength shift from a change of the quantum confinement energy. We have demonstrated single-mode laser emission on the single-exciton recombination transition in core/shell nanorods with a type-II band offset. The simplicity of the wet-chemical synthesis of the nanorods in combination with the high Q -factors of the spherical silica resonators and the efficiency of the fibre-coupling approach for optical pumping make such hybrid systems excellent candidates for studies of the lasing properties of novel gain media and cavity quantum electrodynamic effects. In addition to the single-excitonic nature of the laser emission, other laser-operating characteristics, such as its single-mode emission, which is associated with low levels of noise, and the ultra-low lasing thresholds that were obtained (thanks to the larger dipole oscillation strength of the antenna-designed nanocrystals), are appealing for quantum information processing. Furthermore, the ability to tune the emission wavelength of these WGM microlasers in the visible spectral range is interesting for applications related to biosensing. Considering the inherent potential of colloidal nanocrystals for hybrid integration onto a wide range of platforms and optical resonators, one could envisage the use of optically or even electrically pumped single-exciton lasers based on specialist nanocrystal designs for integrated photonic, lab-on-a-chip and optical interconnect applications. Advances in the development of colloidal nanocrystalline gain media like the recent demonstration of nearly temperature-insensitive threshold for amplified spontaneous emission from CdSe/CdS quantum core/shell (dot/rod) structures [55] can pave the way for the realization of such miniature integrated sources. Fabrication of silica fibre-optical devices Coupling of pump light to the circumference of microsphere resonators can be realized either with free-space optics or by evanescent wave coupling with the use of channel waveguides in integrated optics configurations, prisms, side-polished fibre couplers and tapered fibres [45] . We adopted the latter method for our experiments and used tapers fabricated by the flame-brushing technique [56] , which involves heating of a section of the fibre with a ‘Ω’-shaped resistive microheater operated at a temperature of ~1,400 °C. The microheater was scanned along the fibre section, while at the same time the two fibre ends were pulled in opposite directions by a pair of computer-controlled translation stages of submicron precision. This method can produce taper transitions of well-defined length and shape, and extremely uniform waists, with submicron diameters by controlling the heating and stretching speed. The tapers used had adiabatic transitions to preserve the low propagation loss inherent to the fundamental fibre mode. The microspheres were produced by thermal processing of a fibre taper (stem) by a CO 2 laser beam. Tapers enabled fabrication of microspheres with diameters considerably smaller than the fibre outer diameter, and were drawn from standard telecom silica fibres (outer diameter=125 μm) following the process described in the previous paragraph. The uniform waist-tapered region formed was cut in its centre and then one of the taper ends was heated by the CO 2 laser beam to a temperature in excess of 1,000 °C, causing it to reflow and mould into a spherical-shaped structure due to surface tension. Thanks to the high viscosity of the silica glass, the reflowed structure was highly spherical and extremely uniform, with intrinsically very low surface roughness and, hence, very low scattering loss. After the fabrication process had been completed, they remained attached to their stems, which did not affect the optical modes near the equatorial plane that were excited to produce laser emission. The fibre tips were manufactured using a commercial micropipette puller, in which the heating source was a CO 2 laser, and the pulling process was controlled by a microprocessor. The device enabled fabrication of tips with tapered transition lengths between 1 and 2 mm, and a diameter as small as 40 nm, from fibres with an outer diameter of 125 μm. The taper angle of the tip was designed to be small enough to adiabatically convert the fundamental mode in the fibre core into a fundamental mode guided by the cladding/air interface allowing for transmissions larger than 98%. Calculation of laser energies for the single-exciton and bi-exciton transitions In the single-exciton case, the carrier wavefunctions were calculated from the Schrödinger equations: where ħ is the reduced Plank constant, and are the effective masses of the electron and hole, respectively, which are material dependent ( and for the CdSe core, and and [57] , [58] for the CdS shell), q e , E e , q h and E h are the charges and energy eigenvalues of the electrons and the holes, whereas V cb and V vb are the potentials of the CB and VB, respectively. Finally, in equations (8) and (9), φ e , and φ h represent the electric potentials of the electron and hole, respectively, which account for the Coulombic electron–hole interaction and were calculated from the Poisson equations: here, ρ e and ρ h stand for the electron and hole distributions in the nanorod, respectively, whereas ε and ε o represent the relative permittivity and the vacuum permittivity, respectively, given by: we note that contributions of the CB and VB to the hole and electron wave-functions, ψ h and ψ e , respectively, were neglected, as CdSe and CdS are wide bandgap semiconductors. The wavefunctions were solved iteratively using a finite element method with sequential variation of the nanorod diameter and the energy offset of the CBs, as well as optimization of φ e , and φ h following the Hartree self-consistent potential approach, to match the single-exciton emission line. For the single exciton, we started by setting in the Schrodinger equation (8) the initial potential to zero on the basis of which ψ e was calculated and introduced into the Poisson equation (10). From the latter, the potential generated by the electron was computed and the value derived was introduced into the Schrodinger equation (9) to calculate the ψ h . The resulting wavefunction was in turn introduced into the Poisson equation (11) to obtain the potential generated by the hole. The derived potential was introduced into the Schrodinger equation (8), which was solved to obtain a new expression for ψ e . This procedure was continued until further iterations left unaltered the carriers’ wavefunctions and potentials. In this case, self-consistency was achieved and the derived values were taken as the actual wavefunctions and potentials, respectively. We stress that although the zero potential chosen to initiate the calculation process may give the impression that the electron–hole interaction was not taken into account, the final carrier potentials were indeed introduced in the calculation through the iteration process followed, providing optimal description of the specific quantum system. The Schrödinger equations used for the bi-exciton are essentially similar to those described above, with the only difference being that the electric potentials generated by all the carriers (that is, the two electrons φ e1 and φ e2 , and the two holes φ h1 and φ h2 ) were considered: The electric potentials in the above equations were derived by the Poisson equations: with ρ e1 , ρ e2 and ρ h1 , ρ h2 being the electron and hole distributions in the nanorod, respectively, that can be derived from: To solve the system of equations (14, 15, 16, 17), we followed a similar iteration process with one implemented for the calculation of the single-exciton laser emission. Hence, we assumed zero potentials for the two holes and the second electron to calculate the wavefunction ψ e1 from the Schrodinger equation (14). The resulting wavefunction was then introduced in equation (22) to obtain the distribution ρ e1 , which was in turn introduced in the corresponding Poisson equation (18) to derive the potential φ e1 . This process was repeated for the other carriers and iterated for each of them until the potentials and wavefunctions produced remained unchanged with further iteration. We emphasize that first the core size and CB offset values used in the bi-exciton-related calculations were the ones utilized to reproduce the laser single-exciton laser emission and, second, the calculations yielded a unique value for the bi-exciton lasing wavelength. The calculations were carried out using the Matlab and Comsol software packages with the latter providing the finite element method to solve the Schrodinger and Poisson equations. Calculation of the temperature rise in the hybrid microsphere An analytical expression for the laser-induced temperature of the hybrid microsphere, which also accounts for the reduction caused by the ambient medium (air), was derived for a fixed, Gaussian-shaped laser beam that was exclusively absorbed by the solid sphere and not by the ambient medium [54] . For this purpose, we solved the heat equation: where D is the thermal diffusivity and I = I o ·(1− R )·exp(− r 2 / w 2 ) is the intensity of the irradiating Gaussian infrared beam with a radius w . The following boundary conditions were applied: (a) The balance of energy fluxes at the interface R = R H : (b) The continuity of temperature at the interface R = R H : with T α and T s being the temperature in the ambient medium and the miscrosphere, respectively. (c) The temperature rise at infinity shall vanish: In the following, we demonstrate the validity of our assumption that the impact of the thin layer of nanocrystals on the temperature of the laser-heated silica sphere is negligible and that both media have effectively the same temperature. For this purpose, we consider the heat transported from the sphere given by: where, h =4 nm is the coating thickness and κ s =1.38 × 10 −3 mW m −1 K −1 is the thermal conductivity of silica. The infrared laser beam radius can be approximated as being equal to the microsphere radius, w = R H =4.6 μm. From equation (30), it can be then derived that the relative change in the surface temperature caused by the nanorod coating is: where κ n =2 × 10 −2 mW m −1 K −1 is the thermal conductivity of the nanorods, for which we assumed to be equal to the corresponding value of the bulk CdS crystal. As κ n is an order of magnitude higher than κ s , it becomes clear that the reduction of the temperature of the microsphere due to the heat transport to the nanocrystal layer is insignificant. Finally, with regard to the term in equation (4), which represents the heat transported from the sphere to the air, the ratio κ α / κ s was derived by considering that the heat originating from the hybrid sphere is shared with the air, implying that the fluxes from the sphere ( J s ) and the air ( J a ) should satisfy the equation: where I is the intensity of the infrared light. How to cite this article: Grivas, C. et al. Single-mode tunable laser emission in the single-exciton regime from colloidal nanocrystals. Nat. Commun. 4:2376 doi: 10.1038/ncomms3376 (2013).